Tailless and Atrophin controlDrosophilaaggression by regulating neuropeptide signalling in thepars intercerebralis Aggressive behaviour is widespread throughout the animal kingdom. However, its mechanisms are poorly understood, and the degree of molecular conservation between distantly related species is unknown. Here we show that knockdown of tailless ( tll ) increases aggression in Drosophila , similar to the effect of its mouse orthologue Nr2e1 . Tll localizes to the adult pars intercerebralis ( PI ), which shows similarity to the mammalian hypothalamus. Knockdown of tll in the PI is sufficient to increase aggression and is rescued by co-expressing human NR2E1 . Knockdown of Atrophin , a Tll co-repressor, also increases aggression, and both proteins physically interact in the PI . tll knockdown-induced aggression is fully suppressed by blocking neuropeptide processing or release from the PI . In addition, genetically activating PI neurons increases aggression, mimicking the aggression-inducing effect of hypothalamic stimulation. Together, our results suggest that a transcriptional control module regulates neuropeptide signalling from the neurosecretory cells of the brain to control aggressive behaviour. Aggression is a complex social behaviour that is pervasive across the animal kingdom and has important societal consequences [1] . For many species, aggressive behaviour is important for the acquisition of resources, such as food, territory and mates; however, the behaviour can be energetically costly and can result in damage to the organism. The elucidation of the genes and neuronal circuitry that regulate aggression is key to the understanding of its mechanisms. The fruit fly Drosophila melanogaster has recently emerged as a model system to study aggression [2] , [3] , [4] , [5] , [6] , [7] , [8] , [9] , [10] , [11] , [12] . Several conserved neuromodulators have been shown to play a role in fly aggression [5] , [6] , [7] . For example, serotonin plays a critical role in the modulation of aggression across a broad range of species but the effect is different in vertebrates and invertebrates [13] , [14] . In addition, fly-specific pheromonal cues have been identified that affect aggression in Drosophila [10] , [11] , [12] . What remains unclear is whether the molecular mechanisms that control aggression in flies are mechanistically conserved with those in mammals. Transcriptional control modules that consist of transcription factors, their co-factors, DNA-binding sites and target genes are often conserved in the control of developmental and behavioural processes across a broad range of species [15] , [16] . Such transcription modules are therefore ideal to investigate the question of evolutionary conservation of molecular control mechanisms of specific phenotypes. A classical example in behaviour is the transcriptional negative feedback loop that controls circadian behaviour in most animal species [16] . Circadian mutants were first isolated in a screen for Drosophila eclosion rhythm [17] , and the molecular clock was elucidated in the following decades [16] and found to be remarkably conserved across many species [18] . In mice, a transcription factor, called Nr2e1 or Tlx, was identified almost 20 years ago as having a major effect on aggressive behaviour [19] . Nr2e1 is a transcriptional repressor that belongs to the family of orphan nuclear receptors [20] , [21] and is an orthologue of Drosophila tailless ( tll ), which is critical for early embryonic development [22] , [23] . Mammalian Nr2e1 and Drosophila Tll have a conserved binding site [24] and share a conserved co-repressor [25] , encoded by the Atrophin locus. In addition, some of the known targets are conserved between mice and flies [26] . A deletion of the mouse gene causes abnormal brain development and extreme aggression [19] , [27] , [28] , [29] . These phenotypes are rescued with a human transgene covering the human genomic locus demonstrating molecular conservation between mice and humans even at the level of the regulatory regions of this locus [29] . In addition, single nucleotide polymorphisms in the human NR2E1 locus have been associated with schizophrenia, bipolar disorder and psychopathy [30] —three human disorders associated with excessive aggressive tendencies. However, the mechanism of action of this gene with respect to its extreme aggression phenotype is still not well understood. Here we show that pan-neuronal knockdown of tailless in Drosophila induces a strong aggression phenotype similar to what is observed in mice, and that adult-specific knockdown is sufficient to cause the phenotype. In the adult fly brain, Tailless localizes to the neurosecretory cells of the pars intercerebralis ( PI ), a brain region with functional, developmental and structural similarities to the mammalian hypothalamus [31] . Knockdown of tll specifically in the PI causes aggression and can be rescued by co-expression of human NR2E1. Knockdown of Atrophin ( Atro ), which encodes a co-repressor of Tll, also increased aggression. We further show that Tll and Atro physically interact in vitro and in transgenic animals expressing tagged variants of the two proteins. To explore the role of the PI neurons in the regulation of aggression, we genetically activated these neurons by expressing the bacterial sodium channel, NaChBac [32] . Flies with genetically activated PI neurons show an increased aggression phenotype, similar to electrical stimulation of the mammalian hypothalamus, which also induces aggression in a wide range of mammalian species [33] , [34] , [35] . To characterize the neuronal mechanism of tll knockdown-induced aggression, we blocked neuropeptide processing and release from these neurons and fully suppressed the aggression phenotype. Finally, we show that knockdown of tll in the PI leads to increased release of a neuropeptide reporter, suggesting that Tll controls aggression by regulating the release of neuropeptides from the neurosecretory cells of the PI . Taken together, our results suggest that Tll is part of a transcriptional module that controls aggression in the neurosecretory cells of the pars interecerebralis by regulating the release of neuropeptides. Knockdown of tailless in adult males increases aggression We first asked whether transcriptional control of aggression is conserved between fruit flies and mice and focused on the role of the orphan nuclear receptor orthologue of Nr2e1 in this complex behaviour. In mice, a deletion of the Nr2e1 locus results in brain developmental defects and extreme aggression, although it is not known whether the developmental and behavioural effects are directly linked [19] , [27] , [28] , [29] . The Drosophila genome harbours two Nr2e1 orthologues [20] , [21] , tailless ( tll ) and dissatisfaction ( dsf ) ( Supplementary Fig. 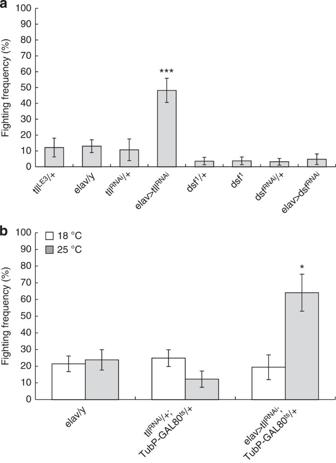Figure 1: Knockdown oftllin the adult fly increases aggression. (a) Fighting frequencies of flies of the following genotypes:tllLe3/+,elav-GAL4/+,UAS-tllRNAi/+,elav-GAL4;UAS-tllRNAi,dsf1/+,dsf1,dsfRNAi/+ andelav-GAL4;UAS-dsfRNAi. Onlyelav>tllRNAimales have significantly higher median fighting frequencies (Kruskal–Wallis ANOVA, ***P<0.001,n=minimum of 70 pairs for each genotype). (b) Fighting frequencies ofelav-GAL4>UAS-tllRNAiin aTubP-GAL80tsbackground and control lines containing only one component of the binary expression system (elav-GAL4/+ andTubP-GAL80ts/+; UAS-tllRNAi/+). All flies were reared at 25 °C and on the day of eclosion were either moved to 18 °C (open bars) or maintained at 25 °C (grey bars) for 7 days. Only elav>tllRNAi; TubP-GAL80tsmales that were maintained at 25 °C after eclosion had significantly higher median fighting frequencies (Kruskal–Wallis ANOVA, *P=0.025,n=minimum of 60 pairs for each genotype). Bar graphs are presented as means±s.e.m. 1 and Supplementary Table 1 ). Null mutations in tll are embryonic lethal [22] , [23] . In contrast, null mutations in dsf are adult viable and have male courtship defects [36] . We analysed existing null alleles of tll ( tll LE3 /+) and dsf ( dsf 1 ) but neither showed an increase in aggressive behaviour ( Fig. 1a ). We also knocked down both genes using RNA interference (RNAi) and assayed for aggression [37] . We used the GAL4/UAS system [38] to drive RNAi alleles, which have been inserted in the same genomic locus [39] . Using the pan-neuronal driver, elav-GAL4 (ref. 40 ), only males in which tll was knocked down showed significantly increased fighting frequencies compared with control animals ( Fig. 1a , Kruskal–Wallis analysis of variance (ANOVA), P< 0.001). Knockdown was verified using western blotting, which shows that Tll levels are significantly reduced in the brains of the knockdown males ( Supplementary Fig. 2 ). These results suggest that tll , but not its paralogue dsf , plays a role in aggression. Figure 1: Knockdown of tll in the adult fly increases aggression. ( a ) Fighting frequencies of flies of the following genotypes: tll Le3 /+, elav-GAL4 /+, UAS-tll RNAi /+, elav-GAL4 ; UAS-tll RNAi , dsf 1 /+, dsf 1 , dsf RNAi /+ and elav-GAL4 ; UAS-dsf RNAi . Only elav>tll RNAi males have significantly higher median fighting frequencies (Kruskal–Wallis ANOVA, *** P <0.001, n =minimum of 70 pairs for each genotype). ( b ) Fighting frequencies of elav-GAL4>UAS-tll RNAi in a TubP-GAL80 ts background and control lines containing only one component of the binary expression system ( elav-GAL4 /+ and TubP-GAL80 ts /+; UAS-tll RNAi /+). All flies were reared at 25 °C and on the day of eclosion were either moved to 18 °C (open bars) or maintained at 25 °C (grey bars) for 7 days. Only e lav>tll RNAi ; TubP-GAL80 ts males that were maintained at 25 °C after eclosion had significantly higher median fighting frequencies (Kruskal–Wallis ANOVA, * P =0.025, n =minimum of 60 pairs for each genotype). Bar graphs are presented as means±s.e.m. Full size image Loss of Nr2e1 in mice causes abnormal brain development in addition to extreme aggression [19] , [27] , [28] , [29] . However, it is unclear whether these brain defects cause the aggression phenotype in mice or whether the behavioural abnormalities are independent from the developmental defects. In flies, we found no obvious anatomical defects in aggressive elav-GAL4>tll RNAi male brains when we immunostained with the neuropil marker Dlg. To address whether the behavioural phenotype in elav-GAL4>tll RNAi males is indeed due to a post-developmental role of Tll, we tested adult-specific knockdown of tll using the TARGET system [41] . This system adds temporal control to the GAL4/UAS system by using an ubiquitously expressed temperature-sensitive GAL4 inhibitor, TubP-GAL80 ts , to block GAL4-induced activation at the permissive temperature (18 °C) and allowing GAL4 induction at the restrictive temperature (25–30 °C) [41] . Only the elav-GAL4>UAS-tll RNAi ; TubP-GAL80 ts flies reared and maintained at 25 °C ( Fig. 1b , Kruskal–Wallis ANOVA, P= 0.0246) or reared at 18 °C and shifted to 25 °C after eclosion ( Supplementary Fig. 3 ) showed significantly increased fighting frequencies compared with the control animals, indicating that adult knockdown is necessary and sufficient to increase aggression. Tll localizes to the adult PI The adult-specific behavioural effects of tll knockdown prompted us to investigate Tll protein localization in the adult fly brain. We performed immunohistochemistry using two different antibodies, one raised against Drosophila Tll [42] and one raised against human NR2E1 (Sigma) that is specific to the highly conserved 50 amino-terminal residues (76% identical to fly Tll). Both antibodies revealed localization of Tll in the PI ( Fig. 2a,b and Supplementary Fig. 4 ), a brain region composed of ~200 neurosecretory cells that has been suggested to be functionally equivalent to the hypothalamus based on molecular, structural and developmental data [31] . Interestingly, mouse Nr2e1 is expressed in the adult hypothalamus [28] , which is known for its important regulatory role in mammalian aggression [43] , [44] . To confirm that the signal observed in the PI was specific to Tll and not to its paralogue, Dsf, we immunostained flies in which the dsf locus is deleted. The signal in the PI was indistinguishable from wild-type and heterozygous animals ( Supplementary Fig. 4 ), further confirming that Tll is expressed in the PI . 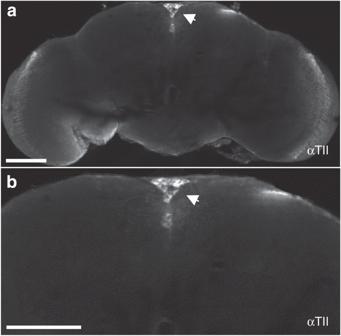Figure 2: Tll localizes to the adultpars ntercererbralis. (a,b) Immunofluorescence image of a wild-type adult brain with anti-Tll antibody. Tll localizes to thepars intercerebralis(arrowhead). Some staining is also observed in the optic lobes. (b) Close-up view of the staining in thePI. Scale bar=100 μm. Figure 2: Tll localizes to the adult pars ntercererbralis . ( a , b ) Immunofluorescence image of a wild-type adult brain with anti-Tll antibody. Tll localizes to the pars intercerebralis (arrowhead). Some staining is also observed in the optic lobes. ( b ) Close-up view of the staining in the PI . Scale bar=100 μm. Full size image PI -specific knockdown of tll induces aggression To assess whether Tll expression in the PI plays a critical role in aggression, we used three GAL4 driver lines ( c929 (ref. 45 ), 50Y (ref. 46 ), dIlp2 (ref. 47 )) with overlapping expression in the PI ( Fig. 3a–c ) to drive tll RNAi specifically in these neurons. Males derived from these crosses displayed significantly increased fighting frequencies ( Fig. 3d , Kruskal–Wallis ANOVA, P<0.001 ). In contrast, we did not observe increased aggression when we used GAL4 drivers to knockdown tll in the eye, central complex or circadian LNv neurons ( Fig. 3d ). These results suggest that Tll affects aggression by acting in the PI neurons. To exclude the possibility that the effect of Tll on aggression is due to expression outside the brain, we blocked GAL4 expression in areas below the head using tsh-GAL80 (ref. 48 ) and found no change in fighting frequencies ( Fig. 3e ). However, when we blocked 50Y-GAL4 with a ubiquitously expressed TubP-GAL80 or a pan-neuronally expressed elav-GAL80 (ref. 49 ), we observed complete suppression of tll knockdown-induced aggression ( Fig. 3e , Kruskal–Wallis ANOVA, P< 0.001). To further show that this effect is due to the specific knockdown of tll, we tested a second RNAi line directed against tll [50] and found a similar increase in aggression when we drove it in PI neurons ( Supplementary Fig. 5 ). We also performed a rescue experiment by co-expressing fly UAS-tll and human UAS-NR2E1 with tll RNAi in the PI . We observed strong suppression of the fighting frequencies in the rescued males (black bars, 50Y>UAS-tll; tll RNAi and 50Y>UAS-NR2E1; tll RNAi ) compared with tll knockdown males ( 50Y>tll RNAi ) ( Fig. 3f , Kruskal–Wallis ANOVA, P< 0.001). These results indicate that the increased aggression phenotype caused by tll knockdown in the PI is specific to tll and that the human gene can functionally substitute for the fly gene in its behavioural regulation. As the PI has been implicated in other behaviours, we also tested whether PI -specific knockdown of tll affected courtship, mating and locomoter activity ( Supplementary Fig. 6 ). We observed no differences in courtship and mating behaviour between the tll knockdown males and their controls; however, we did found a significant decrease in activity in the knockdown males ( Supplementary Fig. 6d , ANOVA, P< 0.01). It has been previously argued that aggressive behaviour read-outs should be adjusted for activity in flies because increased activity is associated with increased aggression [6] . Given that the tll knockdown males have decreased activity, that interpretation would suggest that we may be underestimating aggression in the tll knockdown males. 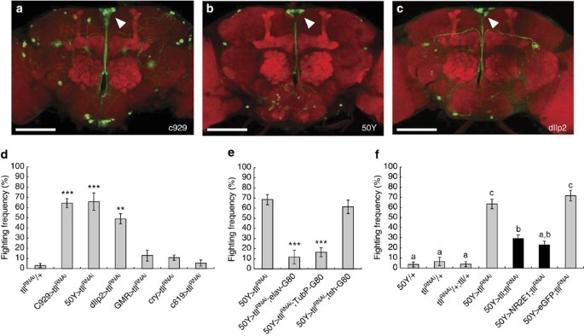Figure 3: Knockdown oftaillessin thepars intercerebralisincreases aggression. (a–c) The GAL4 expression patterns, detected byUAS-eGFP(green), in the adult brain of three different drivers that primarily express in thepars intercerebralis: (a)c929-GAL4, (b)50Y-GAL4and (c)dIlp2-GAL4. Neuropil is marked with an anti-Dlg antibody (red). Arrowheads denote thepars intercerebralis. Scale bar=100 μm. (d) Fighting frequencies of flies expressingUAS-tllRNAiin different regions of the fly brain usingc929-GAL4,50Y-GAL4,dIlp2-GAL4,GMR-GAL4,cry-GAL4andc819-GAL4and a control line ofUAS-tllRNAi/+. Onlyc929>tllRNAi,50Y>tllRNAianddIlp2>tllRNAimales showed statistically significantly higher median fighting frequencies (Kruskal–Wallis ANOVA, **P<0.01 and ***P<0.001,n=minimum of 70 pairs for each genotype). (e) Fighting frequencies of flies withtaillessknocked down in50Yneurons or of flies co-expressingtsh-GAL80,elav-GAL80orTubP-GAL80(GAL80abbreviated as G80). Asterisks denote statistically significant rescue inelav-GAL80andTubP-GAL80co-expressing males (Kruskal–Wallis ANOVA, ***P<0.001,n=minimum of 60 pairs for each genotype). (f) Fighting frequencies of flies withtaillessknocked down in50Yneurons and control lines of flies expressing a component of theGAL4/UASsystem. Fighting frequencies of flies co-expressingtllRNAiand either flytllor humanNR2E1andeGFPin50Yneurons and control lines expressing only one component of theGAL4/UASsystem. Letters denote groups with statistically significant different median fighting frequencies. Black bars show statistically significant rescue in males co-expressingUAS-TllorUAS-NR2E1compared with50Y>tllRNAiand50Y>tllRNAimales co-expressingUAS-eGFP(Kruskal–Wallis ANOVA,n=minimum of 70 pairs for each genotype). Bar graphs represent means±s.e.m. Figure 3: Knockdown of tailless in the pars intercerebralis increases aggression. ( a – c ) The GAL4 expression patterns, detected by UAS-eGFP (green), in the adult brain of three different drivers that primarily express in the pars intercerebralis : ( a ) c929-GAL4 , ( b ) 50Y-GAL4 and ( c ) dIlp2-GAL4 . Neuropil is marked with an anti-Dlg antibody (red). Arrowheads denote the pars intercerebralis . Scale bar=100 μm. ( d ) Fighting frequencies of flies expressing UAS-tll RNAi in different regions of the fly brain using c929-GAL4 , 50Y-GAL4 , dIlp2-GAL4 , GMR-GAL4 , cry-GAL4 and c819-GAL4 and a control line of UAS-tll RNAi /+. Only c929>tll RNAi , 50Y>tll RNAi and dIlp2>tll RNAi males showed statistically significantly higher median fighting frequencies (Kruskal–Wallis ANOVA, ** P< 0.01 and *** P <0.001, n =minimum of 70 pairs for each genotype). ( e ) Fighting frequencies of flies with tailless knocked down in 50Y neurons or of flies co-expressing tsh-GAL80 , elav-GAL80 or TubP-GAL80 ( GAL80 abbreviated as G80). Asterisks denote statistically significant rescue in elav-GAL80 and TubP-GAL80 co-expressing males (Kruskal–Wallis ANOVA, *** P <0.001, n =minimum of 60 pairs for each genotype). ( f ) Fighting frequencies of flies with tailless knocked down in 50Y neurons and control lines of flies expressing a component of the GAL4 / UAS system. Fighting frequencies of flies co-expressing tll RNAi and either fly tll or human NR2E1 and eGFP in 50Y neurons and control lines expressing only one component of the GAL4/UAS system. Letters denote groups with statistically significant different median fighting frequencies. Black bars show statistically significant rescue in males co-expressing UAS-Tll or UAS-NR2E1 compared with 50Y>tll RNAi and 50Y>tll RNAi males co-expressing UAS-eGFP (Kruskal–Wallis ANOVA, n =minimum of 70 pairs for each genotype). Bar graphs represent means±s.e.m. Full size image Tll interacts with Atro to regulate aggression Tll is a known transcriptional repressor and has evolutionarily conserved co-repressors in flies and mice [25] . We tested whether loss of two previously described Tll co-repressors, Scribbler (Sbb) [51] and Atrophin (Atro) [52] , also affect aggression. Similar to tll , both genes are embryonic lethal, and we therefore used RNAi to silence them and assayed for aggression. We found that 50Y>sbb RNAi males did not show significantly increased fighting frequencies, while 50Y>Atro RNAi males did ( Fig. 4a , Kruskal–Wallis ANOVA, P< 0.001). We also knocked down Atro with another previously validated RNAi allele ( Atro IR ) [52] , and again observed a significant increase in fighting frequency compared with controls ( Fig. 4a , Kruskal–Wallis ANOVA, P< 0.01). Pan-neuronal knockdown with Atro IR significantly decreases the level of Atro ( Supplementary Fig. 7 ). Consistent with the stronger behavioural effect of Atro RNAi expression in the PI , elav-GAL4>Atro RNAi flies were lethal and could not be evaluated for knockdown efficiency. We next determined Atro localization and found that it is ubiquitous throughout the brain including the PI neurons ( Fig. 4b and Supplementary Fig. 8 ). To evaluate whether Tll and Atro may act in the same pathway, we used a genetic and cell biological approach. We simultaneously silenced tll and Atro by driving tll RNAi and Atro IR in the PI neurons and found that the double knockdown animals showed the same level of aggression as the single knockdown 50Y>tll RNAi males ( Fig. 4c , Kruskal–Wallis ANOVA, P< 0.001). Although neither is a null allele, the data suggest that Tll and Atro work together to affect aggression rather than in parallel pathways. To examine whether Tll and Atro physically interact, we performed bimolecular fluorescent complementation [53] . We tagged tll with the C-terminal portion of yellow fluorescent protein (YFP) and tagged the C-terminal part of Atro that was shown to interact with Tll in vitro [54] with the N-terminal portion of YFP. We first transfected both constructs in Drosophila S2 cells and observed nuclear YFP signal only when we expressed both constructs together ( Fig. 5j ,n compared to b,f and Supplementary Fig. 9 ). We next made transgenic lines expressing both constructs from an UAS promoter and we observed YFP signal in the PI also only when we expressed both construct simultaneously with the 50Y driver ( Fig. 6a–c and Supplementary Fig. 10 ). Together, these results suggest that Tll and Atro function together to regulate aggression through the neurosecretory cells of the PI . 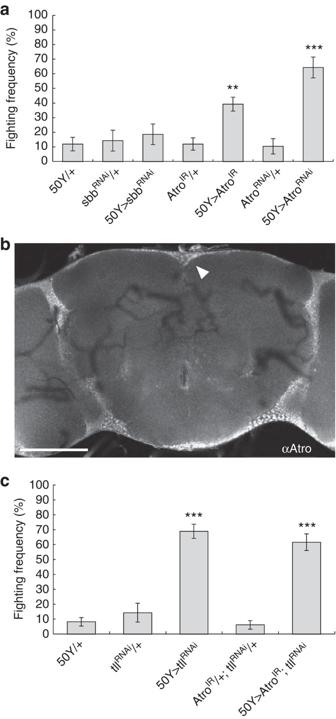Figure 4: Knockdown ofAtrophinin thePIpromotes aggressive behaviour. (a) Fighting frequencies of flies withsbboratroknocked down in thePIusing the50Ydriver and control lines containing only one component of the binary expression system. Only50Y>AtroIRand50Y>AtroRNAiflies have significantly increased fighting frequencies (Kruskal–Wallis ANOVA, **P<0.01 and ***P<0.001,n=minimum of 70 pairs for each genotype). (b) Immunofluorescence image of a slice of an adult male brain stained with anti-Atro antibody. ThePIis indicated with a white arrowhead. Scale bar=100 μm. (c) Fighting frequencies of flies in whichtllalone is knocked down, in whichtllandatroare simultaneously knocked down in thepars intercerebralisusing the50Ydriver, and control lines containing only one component of the GAL4/UAS system. Asterisks denote statistically significant higher medians in thetllandtll/Atroknockdown males compared with the single binary component controls (Kruskal–Wallis ANOVA, ***P<0.001, n=minimum of 60 pairs for each genotype). Bar graphs represent means±s.e.m. Figure 4: Knockdown of Atrophin in the PI promotes aggressive behaviour. ( a ) Fighting frequencies of flies with sbb or atro knocked down in the PI using the 50Y driver and control lines containing only one component of the binary expression system. Only 50Y > Atro IR and 50Y>Atro RNAi flies have significantly increased fighting frequencies (Kruskal–Wallis ANOVA, ** P< 0.01 and *** P< 0.001, n =minimum of 70 pairs for each genotype). ( b ) Immunofluorescence image of a slice of an adult male brain stained with anti-Atro antibody. The PI is indicated with a white arrowhead. Scale bar=100 μm. ( c ) Fighting frequencies of flies in which tll alone is knocked down, in which tll and atro are simultaneously knocked down in the pars intercerebralis using the 50Y driver, and control lines containing only one component of the GAL4/UAS system. Asterisks denote statistically significant higher medians in the tll and tll / Atro knockdown males compared with the single binary component controls (Kruskal–Wallis ANOVA, *** P< 0.001, n=minimum of 60 pairs for each genotype). Bar graphs represent means±s.e.m. 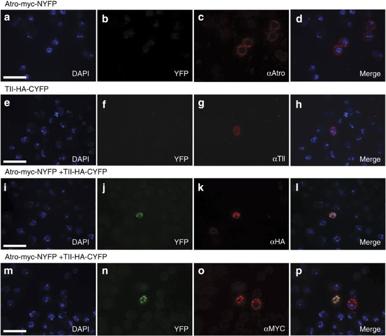Figure 5: Atrophin interacts with Tll in the nucleus in S2 cells. (a–d) Transfection of a single bimolecular fluorescent complementation (BiFC) component, NYFP-MYC-tagged Atro, into S2 cells shows no YFP signal (b) in transfected cells that stain for MYC (c). Red Atro staining labels the cytoplasm, while nuclei are stained in blue with 4′,6-diamidino-2-phenylindole (DAPI) (a). Merged images show red Atro staining around blue nuclei (d). (e–h) Transfection of the other BiFC component, CYFP-HA-tagged Tll, into S2 cells shows no YFP signal (f) in transfected cells that stain for HA (g). Red Tll staining is localized in the nuclei stained in blue with DAPI (e). Merged image shows overlapping signal of red and blue (h). (i–p) Co-transfection of NYFP-MYC-tagged Atro together with CYFP-HA-tagged Tll reconstitutes green YFP signal in the nucleus of co-transfected cells (j,n). Co-transfected cells also stain with an antibody against HA in red (k) or an antibody against MYC in red (o). Red HA signal labels nuclei that are yellow in the merged image (l). Red MYC staining localizes in the cytoplasm and nucleus of co-transfected cell but only in the cytoplasm of cells that only harbour the NYFP-MYC-tagged Atro construct (the lower cell inois not green inn). Merged image shows yellow signal in the nucleus in the upper cell but only red signal in the lower cell (p). Scale bar=20 μm. Full size image Figure 5: Atrophin interacts with Tll in the nucleus in S2 cells. ( a – d ) Transfection of a single bimolecular fluorescent complementation (BiFC) component, NYFP-MYC-tagged Atro, into S2 cells shows no YFP signal ( b ) in transfected cells that stain for MYC ( c ). Red Atro staining labels the cytoplasm, while nuclei are stained in blue with 4′,6-diamidino-2-phenylindole (DAPI) ( a ). Merged images show red Atro staining around blue nuclei ( d ). ( e – h ) Transfection of the other BiFC component, CYFP-HA-tagged Tll, into S2 cells shows no YFP signal ( f ) in transfected cells that stain for HA ( g ). Red Tll staining is localized in the nuclei stained in blue with DAPI ( e ). Merged image shows overlapping signal of red and blue ( h ). ( i – p ) Co-transfection of NYFP-MYC-tagged Atro together with CYFP-HA-tagged Tll reconstitutes green YFP signal in the nucleus of co-transfected cells ( j , n ). Co-transfected cells also stain with an antibody against HA in red ( k ) or an antibody against MYC in red ( o ). Red HA signal labels nuclei that are yellow in the merged image ( l ). Red MYC staining localizes in the cytoplasm and nucleus of co-transfected cell but only in the cytoplasm of cells that only harbour the NYFP-MYC-tagged Atro construct (the lower cell in o is not green in n ). Merged image shows yellow signal in the nucleus in the upper cell but only red signal in the lower cell ( p ). Scale bar=20 μm. 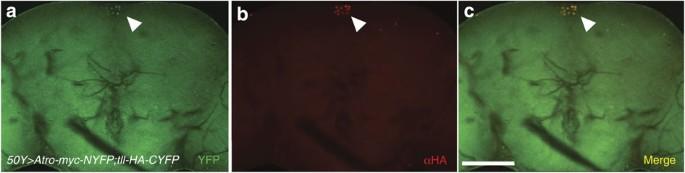Figure 6: Atrophin interacts with Tll in the nucleus in thePI. (a) YFP signal in adult brains of flies co-expressing NYFP-MYC-tagged Atro and CYFP-HA-tagged Tll in thePIwith the 50Y driver. (b) Same brain as inastained with αHA shows CYFP-HA-tagged Tll expression in thePI. (c) Merge between unstained image inaand HA-stained image inb. No signal is observed when only one component of BiFC is expressed (Supplementary Fig. 10). Scale bar=100 μm. Full size image Figure 6: Atrophin interacts with Tll in the nucleus in the PI . ( a ) YFP signal in adult brains of flies co-expressing NYFP-MYC-tagged Atro and CYFP-HA-tagged Tll in the PI with the 50Y driver. ( b ) Same brain as in a stained with αHA shows CYFP-HA-tagged Tll expression in the PI . ( c ) Merge between unstained image in a and HA-stained image in b . No signal is observed when only one component of BiFC is expressed ( Supplementary Fig. 10 ). Scale bar=100 μm. Full size image Tll regulates neuropeptide release from the adult PI Finally, we investigated the underlying neuronal mechanism in the PI that may lead to an increased aggression response in flies. We wondered whether increasing electrical activity in PI neurons may be responsible for the increased aggressive behaviour, similar to the increased aggression phenotype that is observed in mammals when the hypothalamus is electrically or optogenetically stimulated [33] , [34] , [35] , [55] . We expressed the bacterial sodium channel, UAS-NaChBac [32] , to increase electrical activity in PI neurons, and observed a modest but significant increase in aggression in 50Y>UAS-NaChBac males ( Fig. 7a , Kruskal–Wallis ANOVA, P= 0.0059). We observed an even stronger effect when we drove expression of UAS-NaChBac with the dIlp2 driver that is expressed almost exclusively in the PI neurons [47] ( Fig. 3c ) ( Supplementary Fig. 11 , Kruskal–Wallis ANOVA, P< 0.001). Recently, NaChBac expression in the PI was shown to increase neuropeptide release from these neurons [56] , and we therefore tested whether we could block tll knockdown-induced aggression by disrupting neuropeptide function. Neuropeptides that are released from neurosecretory cells typically require processing of precursor forms by the proprotein convertase encoded by amontillado ( amon ) [57] . Following processing, mature peptides are packaged into dense core vesicles, which require the function of Caps (calcium-activated protein for secretion) for subsequent release of these vesicles [58] . When we co-expressed a previously validated RNAi allele directed against amon [57] ( Supplementary Fig. 12 ) together with tll RNAi , we could fully suppress tll knockdown-induced aggression ( Fig. 7b , Kruskal–Wallis ANOVA, P< 0.001). Similarly, a homozygous transposon insertion in Caps fully suppressed the tll knockdown-induced aggression ( Fig. 7c , Kruskal–Wallis ANOVA, P< 0.001). Co-expression of amon RNAi also fully suppressed the NaChBac -mediated activation of the PI neurons ( Supplementary Fig. 11 ). To visualize the effect of tll knockdown on neuropeptide release, we co-expressed a heterologous green-fluorescent protein (GFP)-tagged neuropeptide reporter [59] in the PI . Compared with controls ( Fig. 7d ), GFP staining in the cell bodies of the PI was strongly diminished when we also knocked down tll ( Fig. 7e ). Together with the neuropeptide processing and release suppression results, these staining results suggest that Tll regulates aggressive behaviour through the release of neuropeptides from the PI ( Fig. 7f ). 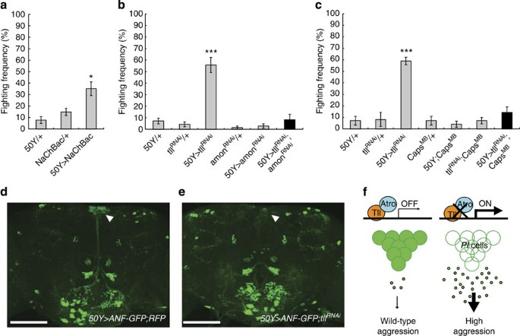Figure 7: Tailless affects aggression through a neuropeptide-based mechanism. (a) Fighting frequencies of flies expressingUAS-NaChBacin thepars intercerebraliswith50Y-GAL4and control lines containing only one component of theGAL4/UASsystem (Kruskal–Wallis ANOVA, *P=0.0059,n=minimum of 90 pairs for each genotype). (b) Fighting frequencies of flies expressingUAS-tllRNAiand/orUAS-amonRNAiin thepars intercerebraliswith50Y-GAL4and control lines containing only one component of the binary expression system. Knockdown oftllin thePIinduces aggression, which is fully suppressed whenamonis simultaneously knocked down (black bar, Kruskal–Wallis ANOVA, ***P<0.001,n=minimum of 60 pairs for each genotype). (c) Fighting frequencies of flies expressingUAS-tllRNAiin thepars intercerebraliswith50Y-GAL4crossed into a homozygous transposon insertion intoCaps,CapsMB03912. Knockdown oftllin thePIinduces aggression, which is fully suppressed by a homozygous mutation inCaps(black bar, Kruskal–Wallis ANOVA, ***P<0.001,n=minimum of 60 pairs for each genotype). (d) Co-expression ofUAS-nRFPand the heterologous neuropeptide reporterUAS-ANF-GFP(the prepro form of atrial natriuretic factor fused to emeraldGFP) inPIneurons with50Y-GAL4shows strong expression in thePIand its projections. (e) Co-expression ofUAS-tllRNAiand the heterologous neuropeptide reporterUAS-ANF-GFPinPIneurons with50Y-GAL4strongly decreases staining in the cell bodies of thePIbut not its projections, suggesting increased release. (f) Schematic diagram depicting the regulation of aggression mediated by a Tailless/Atrophin complex acting in thepars intercerebralison neuropeptide release. Scale bar=100 μm. Figure 7: Tailless affects aggression through a neuropeptide-based mechanism. ( a ) Fighting frequencies of flies expressing UAS-NaChBac in the pars intercerebralis with 50Y-GAL4 and control lines containing only one component of the GAL4/UAS system (Kruskal–Wallis ANOVA, * P= 0.0059, n =minimum of 90 pairs for each genotype). ( b ) Fighting frequencies of flies expressing UAS-tll RNAi and/or UAS-amon RNAi in the pars intercerebralis with 50Y-GAL4 and control lines containing only one component of the binary expression system. Knockdown of tll in the PI induces aggression, which is fully suppressed when amon is simultaneously knocked down (black bar, Kruskal–Wallis ANOVA, *** P< 0.001, n =minimum of 60 pairs for each genotype). ( c ) Fighting frequencies of flies expressing UAS-tll RNAi in the pars intercerebralis with 50Y-GAL4 crossed into a homozygous transposon insertion into Caps , Caps MB03912 . Knockdown of tll in the PI induces aggression, which is fully suppressed by a homozygous mutation in Caps (black bar, Kruskal–Wallis ANOVA, *** P< 0.001, n =minimum of 60 pairs for each genotype). ( d ) Co-expression of UAS-nRFP and the heterologous neuropeptide reporter UAS-ANF-GFP (the prepro form of atrial natriuretic factor fused to emerald GFP ) in PI neurons with 50Y-GAL4 shows strong expression in the PI and its projections. ( e ) Co-expression of UAS-tll RNAi and the heterologous neuropeptide reporter UAS-ANF-GFP in PI neurons with 50Y-GAL4 strongly decreases staining in the cell bodies of the PI but not its projections, suggesting increased release. ( f ) Schematic diagram depicting the regulation of aggression mediated by a Tailless/Atrophin complex acting in the pars intercerebralis on neuropeptide release. Scale bar=100 μm. Full size image We set out to explore whether the molecular mechanisms underlying aggressive behaviour in the fruit fly are conserved with mechanisms that play a role in mammals. We chose to focus our attention on a transcription factor with a strong effect on aggression in mice that has a clear conserved counterpart in Drosophila . Our rationale was based on the idea that conserved transcription modules—which consist of a transcription factor with conserved co-factors, conserved binding site and conserved targets—exist in the evolutionarily conserved control of development [15] and behaviour [16] , [18] . We found that a conserved transcription factor, Tll, and its conserved co-repressor, Atro, indeed affect aggression in flies and that this transcriptional repressor complex acts through a set of adult neurosecretory cells known as the PI , which has remarkable similarity to the mammalian hypothalamus [31] , a brain region known for its critical role in the control of aggressive behaviour in mammals [33] , [34] , [35] , [44] . Moreover, we found that electrical activation of these neurons is sufficient to cause an increase in aggression in flies, just like electrical stimulation of the hypothalamus does in mammals [33] , [34] , [35] . In addition, we were able to block the behavioural effect of PI neuronal activation by blocking neuropeptide processing in these neurosecretory cells. Interestingly, neuropeptide release from the mammalian hypothalamus is also known to play a role in aggressive behaviour [44] . Thus, we have shown that three key mechanisms involved in the control of mammalian aggression are also involved in the control of fly aggression and that they may in fact be a single mechanism. The orphan nuclear receptor Nr2e1 or Tailless is known to have conserved co-repressors [25] , binding sites [24] and targets [26] , and loss of function of this gene in mice has a strong aggression phenotype [19] , [27] , [28] , [29] that can be rescued with a human genomic transgene [29] . The fly harbours two Nr2e1 orthologues [20] , [21] , tailless ( tll ) and dissatisfaction ( dsf ), the former best known for its essential role in early embryogenesis [22] , [23] the latter known for its effect on courtship [37] . When we knocked down tll , we observed a strong aggression phenotype similar to the phenotype observed in mice, while we found no effect in dsf mutants. In mice, loss of Nr2e1 also causes severe brain defects [19] , [27] , [28] , [29] but it is unknown whether these developmental brain abnormalities are required for the extreme behavioural response. We show that adult-specific knockdown of tll is sufficient to cause aggression, thereby uncoupling the developmental and behavioural defects. It will be interesting to examine whether this adult role of Tll holds true in mice. To further test the idea of a conserved transcription module controlling aggressive behaviour, we also examined the role of a known co-factor of Tll. We found that knockdown of a conserved co-repressor of Tll in mice and flies [25] , encoded by the Atrophin locus, also caused an increase in aggression. Drosophila Atro (also known as Grunge ( Gug )) shows similarity to two mouse paralogues [25] , atrophin 1 ( atn1 ) and atrophin 2 ( atn2 , also known as Rere ). A knockout allele of the former has no obvious phenotypic effects [60] , while a null allele of the latter is embryonic lethal [61] . A polyQ expansion of human atn1 causes a dominant neurodegenerative disease, called dentatorubral pallidoluysian atrophy [62] , [63] . Patients with this disease develop neurodegenerative symptoms as well as psychiatric problems including excessive aggressive behaviour [64] , in some cases before the onset of neurodegeneration [65] . The mouse model expressing the human mutation recapitulates many of these phenotypes, including excessive aggression [66] . Fly Atro is more similar to atn2/rere than the shorter atn1 gene but contains several stretches of polyQs that are only found in atn1 (ref. 25 ). In mice, Atn1 and Atn2 can dimerize and the expanded polyQ variant of Atn1 binds more strongly to Atn2 (ref. 67 ). It is intriguing to speculate that excessive aggression in patients with dentatorubral pallidoluysian atrophy may involve a transcriptional module affecting the function of an NR2E1/ATN2 repressor complex in the hypothalamus. To further explore the cellular mechanism of action of Tll, we investigated its expression pattern and found strong expression of Tll in the neurosecretory region of the PI . These neurons have been suggested to be part of an ancient neuro-endocrine axis shared between vertebrates and invertebrates [68] . Multiple lines of evidence have suggested that the PI–corpora cardiaca system has structural, developmental and functional similarities with the mammalian hypothalamic-pituitary axis [31] , [68] . Electrical and optogenetic stimulation of the mammalian hypothalamus leads to a strong increase in aggression in a wide range of mammalian species [33] , [34] , [35] . Release of neuropeptides from the mammalian hypothalamus also plays an important role in aggression [44] . On the basis of these two mammalian mechanisms involved in aggression and the known similarity between these neurosecretory neuronal anatomies in mammals and flies, the Drosophila PI is an excellent candidate for a role in aggression regulation. When we knocked down tll in the PI neurons, we observed a strong increase in aggression that we could rescue by co-expressing the human NR2E1 gene, suggesting mechanistic conservation between flies and mammals. If PI neurons are indeed functionally similar to the mammalian hypothalamus in their control of aggressive behaviour, stimulation of these neurons would be predicted to increase aggressive behaviour just as electrical stimulation of the hypothalamus does in mammals. We tested this idea by genetically activating the PI with the bacterial sodium channel, NaChBac, which is known to increase electrical activity in the cells where it is expressed [32] . As expected, we observed an increase in aggression in males with NaChBac-activated PI neurons. Recently, it was shown that NaChBac expression in the PI increases neuropeptide release [56] . When we blocked neuropeptide processing by inhibiting the neuropeptide preproconvertase Amon [57] , we could fully suppress this response. We next explored whether the mechanism of tll knockdown-induced aggression in the PI is similarly based on increased neuronal activation and neuropeptide release from the PI . Indeed, when we blocked neuropeptide processing through Amon function, or neuropeptide release by reducing Caps, which is required for dense core vesicle release [58] , we could fully suppress the tll knockdown-induced aggression response. Finally, we used a heterologous neuropeptide GFP reporter [59] to visualize the effect of tll knockdown on neuropeptide release from PI neurons and showed that the reporter nearly completely vanishes from PI neurons when tll is knocked down. The identity of the specific neuropeptide(s) that regulate aggression through this transcriptional module is currently not known. There are at least 40 different neuropeptide-encoding genes with corresponding receptors in the Drosophila genome [69] , and it will be interesting not only to identify the causative peptide but to show whether it is conserved in mammals and whether it is directly regulated by the Tll/Atro transcriptional repressor complex. The well-established role of Tll as a transcription factor [20] , [21] , [26] , [70] makes it likely that the behavioural effects that we observe are caused by changes in transcription, although we have not identified direct targets of Tll in this novel adult process. However, together our results suggest that Tll and Atro are part of the transcription module that controls the activity of PI neurons affecting the release of neuropeptides that regulate aggressive behaviour. Our findings in flies suggest that three mechanisms that are involved in the regulation of aggression in mammals—transcriptional control by Nr2e1 (refs 19 , 27 , 28 , 29 ), electrical [33] , [34] , [35] or optogenetic [55] stimulation of hypothalamic neurons and neuropeptide release from the neurosecretory cells of the hypothalamus [44] —may in fact be a single mechanism that may represent a core aggression regulatory mechanism in all animals. Fly stocks and rearing conditions The following fly strains were obtained from the Bloomington stock center: UAS-tll JF02537 ( tll RNAi , BL27242); UAS-dsf JF02537 ( dsf RNAi , BL29373); UAS-sbb JF02375 ( sbb RNAi , BL27049); UAS-Atro HMS00756 ( Atro RNAi , BL32961); UAS-EGFP (BL5431); UAS-NaChBac (BL9466); UAS-amon RNAi 78b (BL29009); Caps MB03912 (BL24279); and UAS-preproANF-EMD ( ANF-GFP , BL7001) . tll LE3 was a gift from J. Merriam (University of California, Los Angeles). tll RNAi2 was a gift from Tzumin Lee (Janelia Farm Research Campus, Virginia). Df(2L)clot7 , Df(2L)dsf 3 and dsf 1 were gifts from K. Finley (San Diego State University). c929 and cry-GAL4 were gifts from P. Shaw (Washington University St. Louis Medical School). 50Y was a gift from R. Greenspan (University of California, San Diego). elav-GAL4 c155 and dIlp2-GAL4 were gifts from S. Pletcher (University of Michigan). GMR-GAL4 was a gift from H. Bellenaylor College of Medicine). c819-GAL4 , tubP-Gal80 and tubP-GAL80 ts were gifts from G. Roman (University of Houston). tsh-GAL80 was a gift from G. Miesenbock (Cambridge University). elav-GAL80 was a gift from L. Jan (University of California, San Francisco) and UAS-Atro IR1 was a gift from C.-C. Tsai (University of New Jersey Medical School). All flies were reared on yeast, cornmeal, molasses and agar food at room temperature (22.5±0.5 °C) on a 12-h light/12-h dark cycle. The sequences that are targeted by the different RNAi constructs against tll and Atro are shown in Supplementary Information ( Supplementary Fig. 13 ). Aggression assay All aggression analyses were performed using the arena assay as previously described with minor modifications [37] . Briefly, one pair of 7- to 8-day-old males was introduced into each of the 35 cells of the arena chamber and filmed for 20 min immediately upon loading. All males were collected on the day of eclosion and were isolated 2.5 days before the assay. We typically tested 70 pairs of flies per genotype and the different genotypes were tested side-by-side. In the analysis, we primarily focused on fighting frequency (the percentage of males that establish a clear dominance hierarchy in the 20-min observation interval). Fighting frequencies correlate very well with other aggression parameters such as lunge number [37] . We scored only unambiguous stereotypical fighting actions such as wing threat, charging/lunging, tussling and boxing. Average fighting frequencies from 70 pairs of flies are plotted with s.e.m. Courtship and mating behaviour For courtship analysis, 10 2- to 5-day-old males of each genotype were tested against CantonS control virgin females that were collected on the morning of the experiment. Flies were videotaped for 10 min and all courtship parameters were recorded. Courtship index was calculated as the percentage of courting over the total observation time. Courtship latency was calculated as the time until the first courtship element. For mating parameters, 30 4-day-old males of each genotype were group-mated with 2- to 4-day-old virgin CantonS females. Latency to copulation and total mating duration were measured and averaged for all the pairs. Sleep and activity analysis Sleep and activity data were analysed in trikinetics monitors (TriKinetics). Four-day-old males were loaded into glass tubes, with food on one end, sealed with wax to prevent desiccation of the food and a foam plug on the other end. Tubes were loaded into the monitors and recorded for 4 days using the DAMSystem data acquisition software (TriKinetics), which records how many times a fly crosses an infrared beam throughout the observation period. Rest/activity data were analysed in Excel [3] . Thirty-two males of each genotype were tested for 3 consecutive days after 1 baseline day. All flies were tested between 4 and 8 days of age. Quantitative RT–PCR Twenty larval brains were dissected from Elav-Gal4; UAS-amon7B , Elav-Gal4/Y and UAS-amon7B/+ male larvae. The tissue was homogenized in 1 ml TriZol extraction buffer and RNA-extracted according to the manufacturer’s instructions. Total RNA (500 ng–1 μg) was used to generate cDNA using SuperScript III First-Strand Synthesis Kit and Oligo dT primer. Quantitative RT–PCR (PCR with reverse transcription) was performed using PowerSYBR Green (Applied Biosystems) to amplify amon using the following primer sets Forward 5′-AAGAACACGGGTCAGAATGG-3′ and Reverse 5′-GGATACGGAAAGGGATCGTT-3′. For normalization, rp49 was also quantified using the following primers Forward 5′-ACTCAATGGATACTGCCCAAGA-3′ and Reverse 5′-CAAGGTGTCCCACTAATGCAT-3′. Three biological replicates for each sample were analysed. Results were obtained and quantified using Applied Biosystems 7900 HT machine and SDS 2.3 software. Molecular cloning and transgenic strains Fly tll cDNA was obtained from the BDGP (clone no. IP01133) and was digested with EcoRI and XhoI (NEB), creating a fragment containing the 5′-untranslated region (UTR), open reading frame and 3′-UTR. The open reading frame human NR2E1 was PCR-amplified from a human brain cDNA library (kindly provided by J. Neul, Baylor College of Medicine). The fly tll cDNA and human PCR product were then cloned into pUAST- attB site (kindly provided by K. Venken, Baylor College of Medicine) using EcoRI and XhoI. Bimolecular complementation vectors were obtained from S. Bogdan (University of Munster, Berlin, Germany). Full-length tll was cloned in frame into the HA (haemagglutinin)-CYFP156-239 (ref. 53 ) vector as an EcoRI fragment deleting the stop codon of tll . The C-terminal 870-bp fragment of Atro [9] was cloned in frame downstream of the NYFP1-173-MYC [53] vector as an XhoI–XbaI fragment. Reciprocal constructs were also generated for tll and Atro but they yielded no interaction in vitro in S2 cells. All the constructs were verified by sequence analysis and subsequently injected into fly embryos containing an attP site on the second or third chromosome and a φC31 integrase on the first chromosome (kindly provided by K. Venken, Baylor College of Medicine). Transformants were crossed to a cantonized w ; Gla / CyO (for second chromosome inserts) or w ; Sb / TM6, Tb (for third chromosome inserts) stock to remove the φC31 integrase chromosome and to balance and homozygose the transgene. Immunohistochemistry and western blotting For immunohistochemistry, adult brains were dissected in ice-cold 4% paraformaldehyde–phosphate-buffered saline (PBS) and were further fixed for a total of 60 min. Next, the brains were rinsed quickly three times with PBS-0.5% Triton X-100 (PBT) and then washed three times for 20 min in PBT at room temperature. The brains were then blocked in 5% normal goat serum–PBT for 1 h at room temperature. Samples were incubated in 5% normal goat serum–PBT with primary antibody for two nights at 4 °C. After three 20-min washes with PBT, the brains were incubated in 5% normal goat serum–PBT with secondary antibody for two nights at 4 °C. The brains were then washed four times for 20 min and then overnight at 4 °C. Finally, brains were mounted in SlowFade mounting medium (Invitrogen) and covered with a no. 0 glass coverslip. The immunostained brains were imaged with an inverted Zeiss Confocal Microscope (Axiovert 100 M). The following primary antibodies were used for immunofluorescence: mouse anti-Dlg (1:100; Developmental Studies Hybridoma Bank); rabbit anti-GFP (1:100; Invitrogen) or mouse anti-GFP (1:200; NeuroMab); rabbit anti-Tll [42] (1:100; gift from J. Reinitz, University of Chicago); rabbit anti-human NR2E1 (SAB2101643, 1:100; Sigma); and rabbit anti-Atro [52] (1:2,000; gift from C.-C. Tsai, University of New Jersey Medical School). Mouse anti-HA (16B12, 1:100, Covance) and mouse anti-MYC (9E10, 1:10; Developmental Studies Hybridoma Bank). Alexafluor secondary antibodies were obtained from Invitrogen and were used at a final concentration of 1:500. Images were analysed with AxioVision Software (Version 4.8.2.0, Zeiss) and further processed using Adobe Photoshop CS3 Extended (Version 10.01, Adobe). Western blotting was performed using standard protocols using rabbit anti-NR2E1 (1:1,000; Sigma), rabbit anti-Atro (1:5,000) and rabbit anti-Dlg (1:2,000; Millipore). Horseradish peroxidase-conjugated secondary antibodies were used at a concentration of 1:2,000 (Millipore). Full-length images of western blots are shown in Supplementary Information ( Supplementary Figs 14,15 ). Transfection and immunofluorescence of cultured S2 cells Drosophila S2 cells (1 × 10 6 cells per well) were added to a six-well plate with a 22 × 22 mm glass coverslip in 2 ml of culture media. After 24 h of growth, cells were transfected with the Act5C-GAL4 driver vector and the tll-HA-CYFP and Atro-MYC-NYFP bimolecular fluorescent complementation vectors. Two micrograms of each vector were resuspended in a 100-μl volume to which 3 μl of FuGENE HD Transfection Reagent (Promega) was added and incubated for 15 min at room temperature. The transfection complex was added to the cells with a gentle swirl and left to grow at room temperature. Forty-eight hours post transfection, the coverslips were moved to a new six-well plate for immunofluorescent staining. The cells were fixed in 1 ml of 4% formaldehyde in PBS for 20 min on a gentle shaker at room temperature. The cells were permeabilized and washed twice in 1 ml PBT (1 × PBS with 0.1% (w/v) BSA and 0.1% Triton) for 15 min. All washes were performed at room temperature on a gentle shaker. The cells were then blocked for 1 h at room temperature in 1 ml of PBT with 5% normal goat serum (NGS, Abcam) while shaking followed by incubation with primary antibody in PBT with 5% NGS for 1 h at room temperature by placing the coverslip (cell side down) on 40 μl antibody solution on parafilm. Cells were washed four times for 30 min in PBT. Subsequently, the cells were incubated with secondary antibody for 2 h using the same procedure as for the primary antibodies. Finally, the cells were washed three times for 20 min and mounted in 15 μl Slowfade Gold (Life Technologies) with 1 μl 4′,6-diamidino-2-phenylindole. The immunostained S2 cells were imaged with an Axioplan2 Zeiss microscope equipped with an ApoTome. Images were captured and analysed with AxioVision Software (Version 4.8.2.0, Zeiss) and further processed using Adobe Photoshop CS3 Extended (Version 10.01, Adobe). Statistical analysis Aggression data are typically not normally distributed and for these data medians were statistically compared using the non-parametric Kruskal–Wallis ANOVA for unpaired groups. We used the Mann–Whitney U- test for post hoc comparisons to identify those groups that differed to a statistically significant extent. Mating and courtship and sleep and activity data were analysed by ANOVA. Statistically significantly different groups were identified using Tukey–Kramer post hoc tests. Behavioural data are presented as bar graphs representing the means with s.e.m. How to cite this article: Davis, S. M. et al. Tailless and Atrophin control Drosophila aggression by regulating neuropeptide signalling in the pars intercerebralis . Nat. Commun. 5:3177 doi: 10.1038/ncomms4177 (2014).